78,000-year-old record of Middle and Later Stone Age innovation in an East African tropical forest The Middle to Later Stone Age transition in Africa has been debated as a significant shift in human technological, cultural, and cognitive evolution. However, the majority of research on this transition is currently focused on southern Africa due to a lack of long-term, stratified sites across much of the African continent. Here, we report a 78,000-year-long archeological record from Panga ya Saidi, a cave in the humid coastal forest of Kenya. Following a shift in toolkits ~67,000 years ago, novel symbolic and technological behaviors assemble in a non-unilinear manner. Against a backdrop of a persistent tropical forest-grassland ecotone, localized innovations better characterize the Late Pleistocene of this part of East Africa than alternative emphases on dramatic revolutions or migrations. The terms Middle Stone Age (MSA) and Later Stone Age (LSA) have long been used to frame discussions of behavioral and cultural change in Africa [1] . Changes in lithic production (such as making elongate blades and stone-tipped arrows [2] , [3] ), the appearance of symbolic material culture [4] , [5] , and subsistence diversification [3] associated with the MSA and LSA have all been identified as important thresholds in human cognitive and social evolution [3] , [6] . Many researchers have highlighted the revolutionary nature of MSA and LSA human capacities, in some cases arguing that they reflect cognitive evolutionary developments [7] or that they stimulated pan-African and global migrations from 60,000 years ago (ka) onwards [8] , [9] . On the other hand, recent discoveries in southern Africa have suggested a more gradual development of these material culture traits [10] , [11] , [12] , [13] . The debate as to the significance and tempo of behavioral changes during the MSA and LSA has largely focussed on the temperate and coastal environments of southern Africa [12] , [14] . This is due to a general lack of well-dated, well-stratified records in other key areas of the African continent, particularly across the period 80–40 ka, though the Haua Fteah and Taforalt in North Africa are notable exceptions [15] , [16] . Long-term, dated records from East Africa remain scarce. Several East African sites have produced evidence for novel practices, reflected in the appearance of backed stone tools and beads over the last 60–40,000 years [17] , [18] , [19] , [20] , [21] , [22] . However, the chronologies and environmental contexts of these key behavioral transitions are not clear. Sites >50,000 years old have only just begun to be identified beyond the East Africa Rift System [23] and are limited to the Lake Victoria region [24] , [25] , [26] . The new archeological cave site of Panga ya Saidi (PYS) described here offers an opportunity to address geographical and ecological biases in our understanding of early human behavioral and cultural change. The site is situated 15 km from the present-day shoreline in the Zanzibar-Inhambane coastal forest mosaic that runs along the East African littoral, with the coastal shelf dropping below −125 m depth within 5 km of the modern coastline (Fig. 1a ) (Supplementary Note 1 ). The cave is in the Dzitsoni limestone hills on an ecotone between lowland tropical forest and savannah (SM5). Excavations at PYS have revealed exceptional preservation and stratigraphic integrity, and a record of human activity back to ~78 ka, including a rich technological sequence that includes lithic forms elsewhere associated with the MSA and LSA. Alongside a rich range of paleoecological indicators, these features mean that the site offers a rare opportunity to study human behavioral changes in an evolutionarily critical, but poorly-understood, region of Africa. Fig. 1 Environmental setting and PYS stratigraphic section. a The location of PYS in the tropical moist forest of coastal East Africa, situated in the Ditzoni upland, southeastern Kenya. b The stratigraphic sequence of PYS showing the Layers and modeled ages, with example of a micromorphological thin section, illustrating the rich biogenic/anthropogenic contents in the sediments (Sh shell, Bn bone, Lt lithic, Ch charcoal). Note that Layer 12 was not continuous across the whole excavation and did not occur in this section. Age estimates are shown as the median of the highest posterior density age range for simplicity Full size image Stratigraphy and chronology The 3 m deep excavated sequence at PYS encompasses 19 layers (Supplementary Note 2 ) (Fig. 1b ). Three lithological boundaries divide the profile into four main lithostratigraphic units that are discussed in detail in Supplementary Note 1 . A series of 20 stratigraphically ordered and internally consistent radiocarbon and optically stimulated luminescence (OSL) age estimates, when included in a Bayesian model, show human occupation in every Marine Isotope Stage (MIS), from late MIS5 c. 78 ka into the Holocene (Supplementary Note 3 ). Geoarchaeological and micromorphological studies indicate that the sequence consists of fine colluvia, spalling, and anthropogenic deposits with abundant organic and cultural microremains (e.g., fauna, flora, lithic microdebitage – Supplementary Notes 4 and 5 ). Geomorphological and magnetic susceptibility proxies for human occupation intensity (Fig. 2 ; Supplementary Note 2 ) indicate a pattern of intermittent pulses of human activity. In the early part of the sequence, in Layers 19, 18, and the lower part of Layer 17 (~78–73 ka), occupation intensity is low. This is followed by a possible hiatus when both lithics and charcoal >c. 125 μm drop off, and magnetic susceptibility and biogenic input signals are dramatically reduced (Fig. 2 ). Human occupation proxies subsequently show a general trend of increasing intensity from Layer 16 (beginning ~67 ka) to the Holocene (Fig. 2 ). Fig. 2 Selected artifacts from PYS. a Levallois core from Layer 11. b Two backed lithic artifacts from Layer 11. c Backed lithic artifact from Layer 3. d Notched bone from Layer 8. e Notched bone from Layer 9. f Ocher crayon from Layer 10. g Ostrich eggshell bead from Layer 8. h Conus shell bead from Layer 16. i Gastropod shell bead from Layer 4 Full size image Cultural artifacts The long artifactual sequence is comprised of 17 ocher fragments, eight worked bone artifacts, 88 ostrich eggshell beads, 27 marine shell beads, five exotic manuports, as well as >30,000 knapped stone artifacts, including Levallois cores and backed artifacts—typical of MSA and LSA technologies, respectively [6] , [27] , [28] (Fig. 3 ). The metrics and characteristics of these technologies are discussed in greater detail in Supplementary Note 4 . The possible hiatus or ephemeral occupation in the PYS sequence between 73 and 67 ka corresponds with a change in the stone artifact sequence. In the early part of the sequence stone artifacts are characterized by large flakes (Fig. 2 ), often made using variations of the Levallois method, and large retouched points (Supplementary Note 4 ), comfortably fitting with other contemporary MSA assemblages [29] . Immediately after the hiatus, in Layer 16, there is a shift in rock type proportions from principally microcrystalline limestone to cryptocrystalline quartz and chert, and a concomitant reduction in artifact size (Fig. 2 , Supplementary Note 4 ). Size reduction is evident across all stone artifacts, including within cryptocrystalline materials and retouched tools, demonstrating that this change does not simply reflect variation in procured raw material package size (Supplementary Note 4 ). Fig. 3 The palaeoenvironmental and human occupation proxies from PYS. From left to right: Sedimentology (LM(SC) sandy clayey loam, LM(PS) pebbly sandy loam, LM(PSA) pebbly sandy ashy loam, LM(SA) sandy ashy loam); Depth; Layer divisions; Box and whisker plots of stable oxygen and carbon isotope values of mammalian teeth; Phytoliths, showing the proportion of grass, palm, and woody taxa; Percentage of different bovids in Minimum Number of Individuals (MNI); Terrestrial mollusk rarefied species count; Magnetic susceptibility (XLF and XFD%); Biogenic content of micromorphology thin sections; Microcharcoal abundance; Proportions of selected faunal groups as a percentage of total tetrapod MNI; Lithic density; Lithic material types; Lithic weight (mean debitage weight) Full size image Coupled with the switch to small cryptocrystalline stone tools after ~67 ka is an increased use of bipolar technology (Supplementary Fig. 4 ). A shift in technological emphasis toward bipolar strategies and a reduction in stone tool size is considered a key marker of LSA behavior elsewhere in Africa [27] , [30] , [31] . A change from Levallois to prismatic blade technology and the appearance of backed crescentic tools have also been highlighted as indicators of the LSA [6] , [32] . However, in the PYS sequence, Levallois technology occurs alongside backed crescents in Layers 11 and 12 (~51–48 ka) and Layers 5–3 (~14–1 ka) (Supplementary Note 4 ) (Fig. 3 ). Prismatic blade production is rare in the PYS sequence, but bipolar and Levallois blades become common in the upper part of the sequence (Layers 8–3) (~25–1 ka) (Supplementary Note 4 ). Levallois and bipolar technology, blade production, and backed crescentic tools occur recurrently and intermittently, with no evidence for a unilinear accumulation of traits or a uniform uptake of the latter three traits as a package. Despite changes in technology, stone artifacts remain consistently small and were predominantly produced on cryptocrystalline materials after ~67 ka. Beads, ocher fragments, and worked bone have been associated with behavioral complexity in the Late Pleistocene and occur with increasing regularity through the sequence at PYS (Supplementary Note 4 ). The earliest bead, a Conus sp. shell spire, occurs in Layer 16 which dates from between ~67–63 ka (Fig. 3 ). At ~33 ka (Layer 9) the most common beads were Conus shell spires ( n = 13) (Fig. 3 ). Recurrent engagement with coastal resources for symbolic use is behavioral, rather than geographic, given minimal changes in distance from the shoreline during the site’s occupation (Fig. 1a ) (Supplementary Note 1 ). Ostrich eggshell beads at PYS reach their highest frequency ~25 ka (Layer 8, n = 70), while fully-manufactured beads made of marine shells are the dominant types during the Holocene (Layers 1–5) (Fig. 2 ). Layers 8-10 (~48–25 ka) produced two modified ocher fragments (Fig. 3 ), as well as carved bone and tusk artifacts, including a decorated bone tube (Fig. 3 ) and a small bone point ; artifact types that have been argued to be characteristic of the LSA [28] . In contrast to many revolutionary or unilinear interpretations of technological and cultural development, the PYS sequence reveals a pattern of intermittent presence of different technological traits and symbolic artifacts that have been associated with the MSA and LSA. Paleoecology Numerous proxies point to broad perseverance of tropical forest and grassland environments throughout the sequence (Supplementary Note 5 ). This is indicated, for example, by the consistently high (> 25 species per sample) terrestrial mollusk diversity, with most of the mollusk species requiring humid shady conditions. Sedimentology and magnetic susceptibility data indicates a shift to drier conditions following the early occupation in Layers 17–19 ~78–73 ka (Fig. 2 ) (see also Supplementary Note 5 ). This is supported, albeit with a lag, by the stable isotope data which shows higher stable carbon (δ 13 C) in Layers 10–12 relative to 13–16 and 17 (Supplementary Tables 12 and 13 ), indicative of an increase in the presence of C 4 resources, most likely in the form of grassland, in the diets of fauna being exploited at the site in the region c . 48 ka. Visually, δ 18 O also tracks this trend but there is no statistically significant difference between Layer 17 and Layers 13–16 or Layers 10–12 (Supplementary Tables 14 and 15 ). From ~67–48 ka, paleoenvironmental proxies at PYS show that the local environment underwent relatively little variation until the final occupation of the cave at ~0.5 ka (Fig. 2 ). The wide δ 13 C and δ 18 O ranges of fauna after Layer 17 (Fig. 2 ) (Supplementary Data 1 ) reflects the persistence of C 3 and C 4 vegetation, and a variety of water sources affected to differing extents by evapotranspiration in the vicinity of PYS; likely in the form of a forest-grassland ecotonal setting. A consistent ecotonal situation is supported by zooarchaeological data for the persistent presence of open and bush/forest adapted mammalian species, as well as phytolith datasets that document the continued occurrence of woody, grass, and palm phytoliths in the immediate site environment (Fig. 2 ). The paleoecological datasets from PYS agree with other East African records that point to a period of low amplitude environmental change throughout much of MIS4-1, particularly from records nearer the coast where the maritime influence buffers against temperature extremes [33] , [34] . The consistent presence of the forest-grassland ecotone throughout the last ~67,000 years accompanies evidence for increasing occupation intensity at PYS, perhaps suggesting a growing human presence in the region linked to the use of mosaic habitats. Moreover, alongside the magnetic susceptibility data for increased occupation intensity from 60 ka, this may imply, as has been suggested elsewhere, that the MSA–LSA transition of East Africa is a long-term pattern of change related to growing population densities [33] , [35] . Indeed, the PYS sequence does not document a radical change in technological or cultural behavior in East Africa ~ 60–50 ka that might be suggestive of cognitive or technological “revolutions” or migrations [7] , [8] . Instead, PYS documents a long-term assembly, and intermittent presence, of various innovative traits. In particular, there is no dramatic appearance of an LSA technological package and, instead, older MSA technological traits, such as Levallois cores, exist alongside the development of backed artifacts and blade production. The principal change in the sequence is the reduction in lithic size and the shift to cryptocrystalline materials ~67 ka. From MIS6-3 Homo sapiens began to adapt to a diversity of coastal [13] , [36] , tropical forest [37] , [38] , and hyper-cold [39] , [40] environments across Africa and Eurasia. Humans appear to have adapted locally to these environments, gradually developing new symbolic forms, technological production strategies, and subsistence behaviors. It seems that the Middle and Late Pleistocene of Africa is best characterized by diverse Homo sapiens populations, adopting a range of survival strategies and new forms of social communication on an intermittent, ad hoc basis in different environmental and climatic contexts [41] , [42] . It is this adaptive plasticity that truly defines the expansion and development of humans as a global species. Excavation Our excavation is in a large rockshelter in the first chamber of the collapsed-roof cave, near to the main entrance. Three seasons of excavation between 2010 and 2013 have exposed a 3 m deep sequence, with the trench measuring 3.5 × 2 m at the top stepping into 2 × 1 m at the base. The trenches were excavated using the single context method according to the Museum of London protocols with the addition of total excavated sediment volume recorded for each context. Any animal burrows were excavated by hand and their contents discarded. In situ excavated deposits were dry-sieved on site through a 5 mm mesh. A program of bulk soil sampling for flotation (0.5 mm) and wet-sieving (1 mm) to recover archeobotanical, zooarcheological, and paleoenvironmental microremains was also implemented (see below). Where possible, a minimum sample volume of 60 litres per context was maintained. Smaller contexts (<60 L) were sampled in their entirety. Nineteen stratigraphic layers were identified in the section, each corresponding to a particular excavation context. A continuous column bulk sediment sample was taken for palaeoenvironmental analyses with 100 g samples taken at every 2 cm of depth. Deposits exposed in PYS Trench 4 (2013 excavation) were logged on-site following standard sedimentological procedures [43] , [44] , [45] . Sediment color, texture, composition, structures, postdepositional disturbance and the nature, and geometry of layer boundaries were recorded for each layer resolved by the excavators. Layers were grouped into higher-order, multilayer lithostratigraphic units, as shown in Supplementary Fig. 1 . Micromorphology A set of 23 undisturbed micromorphology sediment samples were collected from the excavated profile in clear polyurethane boxes. In view of the large dimensions and stratigraphic complexity of the excavated trench, sampling was at a reconnaissance scale, concentrating on layer boundaries and distinctive features. Sample boxes were labeled, photographed and plotted on the profile drawing before removal from the profile (Supplementary Fig. 1 ). Out of this sample set, 10 samples from the Pleistocene part of the profile were processed for micromorphological analysis at the Thin Section Micromorphology Laboratory, University of Stirling (sample code PYS; thin sections manufactured by George MacLeod). Samples were air-dried and impregnated with polyester (polylite) resin following standard procedures ( http://www.thin.stir.ac.uk/ ). Ca. 30 μm thick, uncovered, large format thin sections (7.5 × 11 cm) were manufactured from the hardened impregnated blocks. Thin sections were observed with a polarizing microscope at magnifications of ×12.5 to ×400, using plain polarized (PPL), cross-polarized (XPL), and oblique incident light (OIL). Relative abundance of sediment/soil components was estimated using standard semi-quantitative estimation charts [46] , [47] . Key sediment constituents larger than ca. 50 μm (mineral grains; pedoclasts; biogenic particles, etc.) were point-counted using a 0.5 × 0.5 cm grid overlay printed on clear acetate. Point-counted biogenic particles included bone fragments (from small cave vertebrates and larger vertebrate fauna—the latter possibly including human prey); small vertebrate coproliths; indeterminate isotropic particles; shell fragments; charcoal (both woody and non-woody tissue); burnt plant pseudomorphs; ash and ash intraclasts; quartz debitage (Supplementary Fig. 2 ). Paleomagnetism A sub-sample of the continuous column sample from PYS was transported to The Australian Archaeomagnetism Laboratory for preparation and analysis. Once in the laboratory samples were dried to standardize water content, crushed with a non-magnetic mortar, and pestle to become homogenized and then packed into standard 8cc palaeomagnetic plastic cubes. The approach to the analysis follows that of Herries [48] and a number of analyses were run to establish the magnetic mineralogy of the samples. These included mass specific low-field susceptibility (χlf), mass specific high-field susceptibility (χhf), mass specific frequency dependant susceptibility (χfd) and saturation isothermal remanent magnetization acquisition curves and backfields. This was done to understand the mineralogy driving magnetic susceptibility change through identifying ferrimagnetic vs. anti-ferromagnetic minerals on the basis of their coercivity, establish the concentration of magnetic minerals present within each sample, and examine grain size and domain state trends in the sequence. The magnetic susceptibility of each sample was measured using a Bartington MS2 susceptibility-meter connected to an MS2B sensor. Samples were measured at 0.47 kHz (low, χlf) and 4.7 kHz (high, χhf) to attain both low and high frequency susceptibility values. These measurements were then used to compute the frequency dependence of the magnetic susceptibility (χfd) and then expressed as a percentage (χfd%) using the formula stated by Dearing et al. [49] . Isothermal remanent magnetizations (IRM) were induced up to 1 T (representing the saturation IRM: SIRM) using a magnetic measurements pulse magnetizer (MMPM10) and measurements made on an AGICO JR6 magnetometer. Forward-field measurements were taken at 20, 500, 600 mT, and 1 T and back-field measurements at 20, 40, 100, 150, 200, 250, and 300 mT. Full IRM acquisition curves and backfields were also produced for each layer of the site. HIRM measurements were also taken using the method described by Liu et al. [50] . Soft IRM measurements showing the concentration of ferrimagnetic minerals were taken at 20 mT. S-ratios (IRM-300 mT/SIRM and IRM-100 mT/SIRM) were calculated to establish variation in the grain size of ferromagnetic minerals. Remanence of coercivity values were also calculated to further establish the mineralogy, grain size, and domain states of the magnetic minerals present within the samples. Charcoal abundance From the continuous column sample described in SM3, subsamples of 1 cm 3 were extracted for charcoal abundance analysis. The addition of sodium hexametaphosphate to a beaker containing the sample was used to disaggregate the samples and aid in the separation of the organic material and the clay particles [51] . The contents of the beaker was then passed through a 125 μm sieve and the trapped content transferred to a gridded Petri dish. Pieces of charcoal were identified using comparative collections and the total charcoal count was determined through visual inspection and manipulation with a metal probing needle under a Zeiss Stemi 2000-C optical stereomicroscope (×10–40 magnifications). The microscopic charcoal size identified represents charcoal that was locally produced during fires within the catchment area of the site [52] . Radiocarbon dating Items selected for radiocarbon dating were a human bone and a charred sorghum seed (identified by Alison Crowther) from the upper part of the sequence; as well as unidentified charcoal, and ostrich eggshell pieces including a bead, from the middle part of the sequence. These dating samples were either recovered during excavation or taken from the section at the end of excavation. Fourteen 14 C measurements were produced at the Oxford Radiocarbon Accelerator Unit (ORAU) ( n = 10) and by Beta Analytic ( n = 4). Most charcoal samples were prepared using the standard acid–base–acid (ABA) protocol [53] . While for the younger material (<30 ka BP) this is usually sufficient, it has been shown that ABA does not efficiently decontaminate older charcoal samples when compared with the more rigorous protocol: acid–base oxidation/stepped combustion (ABOx-SC) [54] . Paired ABA and ABOx-SC preparation was used on one sample from context 413 C. For this particular sample, ABA and ABOx methodologies produced identical AMS ages. This is probably due to the exceptional state of preservation of the charcoal in this part of the sequence as well as due to the fact that it is not very old sample. For material from lower levels where only ABA dates from Beta Analytic exist these should be considered minimum ages only. This is demonstrated by the much older ages returned from ostrich eggshell samples from similar contexts. It is not possible to interpret radiocarbon ages reliably without calibration, due to variation in the concentration of radiocarbon in the atmosphere through time. All terrestrial 14 C measurements were calibrated using IntCal13 and SHCal13, the most recent internationally agreed calibration curves available [55] , [56] . As PYS lies close to the equator, a 68.2/31.8 northern/southern hemisphere split was used in the calibration curve, taking into account the position of the site relative to the inter-tropical convergence zone. 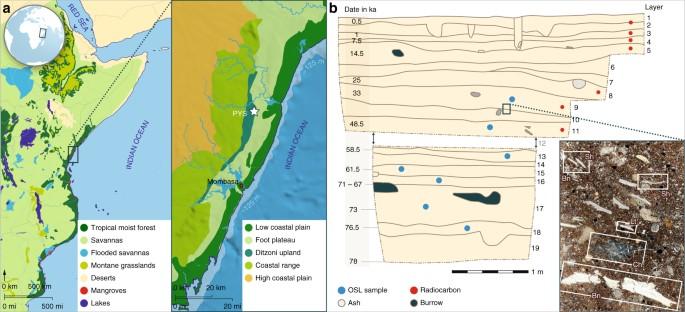Fig. 1 Environmental setting and PYS stratigraphic section.aThe location of PYS in the tropical moist forest of coastal East Africa, situated in the Ditzoni upland, southeastern Kenya.bThe stratigraphic sequence of PYS showing the Layers and modeled ages, with example of a micromorphological thin section, illustrating the rich biogenic/anthropogenic contents in the sediments (Sh shell, Bn bone, Lt lithic, Ch charcoal). Note that Layer 12 was not continuous across the whole excavation and did not occur in this section. Age estimates are shown as the median of the highest posterior density age range for simplicity The radiocarbon ages obtained from PYS are summarized in Supplementary Table 1 . OSL Optically stimulated luminescence (OSL) samples were obtained by hammering metal tubes into section faces following cleaning. The samples were sealed using adhesive tape. Following transport to the Royal Holloway University of London Luminescence Laboratory, samples were processed under subdued orange light. The outer 5 cm of sample (presumed as being exposed to sunlight) was removed and retained for background radioisotope concentration determination. Quartz was extracted from the part of each sample not exposed to sunlight following burial. As the bedrock at PYS is primarily composed of carbonate, samples were initially wet-sieved to isolate the 212–180 µm size fraction. This removes large bedrock clasts from the sample before acid treatment, meaning that the possibility of incorporating grains liberated by dissolution of the bedrock was minimized. The volume of 1 M HCl and H 2 O 2 were used to remove carbonates and organic matter from the 212–180 µm fraction, respectively. The samples were then re-sieved at 180 µm and quartz extracted from the >180 µm fraction using density separations at 2.62 and 2.70 g/cm 3 followed by a HF acid etch (23 M HF for 60 min followed by 10 M HCl rinse). The resulting, etched samples were sieved at 150 µm to remove partially dissolved grains. All samples were then stored in opaque containers prior to measurement. All OSL measurements were carried out using a Risø TL/OSL-DA-15 automated dating system [57] , fitted with a single-grain OSL attachment [58] , [59] . Single-grains were stimulated using a 10 mW Nd: YVO4 solid-state diode-pumped green laser (532 nm) focused to yield a nominal power density of 50 W/cm 2 [57] . All infrared (IR) stimulation was carried out using an IR (870 nm) laser diode array yielding a power density of 132 mW/cm 2 . OSL passed through 7.5 mm of Hoya U-340 filter and was subsequently detected using an Electron Tubes Ltd 9235QB15 photomultiplier tube. Irradiation was carried out using a 40 mCi 90 Sr/90Y beta source providing ~6 Gy/min. This source is calibrated relative to the National Physical Laboratory, Teddington 60Co γ-source (Hotspot 800) [60] . Due to the spatial inhomogeneity of beta emitters across the active face of our 90 Sr/90Y beta source we calibrated the dose rate to each individual grain position on a single-grain disc [61] using the method reported by Armitage et al. [62] . For more detail on measurement and quality criteria see Supplementary Note 3 . Bayesian methods The absolute age determinations were used to construct an age model using Bayesian software (OxCal 4.3 [63] ) and the INTCAL13 curve. The determinations were input as values in fraction modern (fM) plus or minor fM errors at 1σ (R_F14C in OxCal). In order to determine whether there are problematic determinations that do not agree with the prior framework, an outlier detection method was applied. When there is a lack of agreement with the prior framework, significant outlier results allow us to quantify the degree of difference. Values excessively higher than the prior outlier probabilities applied are automatically down-weighted in the models. A posterior outlier probability of 0.5 means that the radiocarbon likelihood of the sample is only included in half of the runs of the model. The two Beta dates were assigned a 0.3 value to reflect the inadequate chemical protocol applied in the decontamination of these samples prior to measurement. Only age estimates older than 20,000 years ago were included in the model. The inclusion of younger ages does not affect the older ages at all. Younger ages were excluded because of the large span of the dates; the model runs with a broad resolution of 50–100 years for the older data, whereas 20 years would be more appropriate for the younger data. In each Bayesian model, a start and end boundary was added in order to bracket the archeological phases within the sequence. The posterior distributions of these boundaries facilitated determination of probability distribution functions (PDF) for the beginning and ending of these phases of activity. Due to the presence of a depositional hiatus represented in the later part of Layer 17, we used two boundaries between the end of 17 and start of Layer 16. In addition, due to uncertainties related to the reliability of sample OSL-7 (see text above) these age estimates were not included in the model. Lithics A total of 30,420 lithic artifacts were recovered through the excavation seasons at PYS between 2010 and 2013. The analyses proceeded by classifying all lithics in accordance with stratigraphic context, raw-material type, and technological class. All artifacts were subsequently weighed and counted according to these categories. Cores and retouched artifacts were further classified in accordance with reduction strategy and typology. For unretouched flakes, blades, Levallois flakes, and bipolar flakes were counted. Levallois [64] , bipolar [65] , laminar, and discoidal strategies as well as resultant blanks were all documented to varying frequencies in a number of the layers. Beads, osseous artifacts, and ocher Over two hundred potential beads, bone tools, engraved bone and stone objects, and pigment lumps recovered during excavation, were examined under a low power reflected light microscope in search for anthropogenic modifications. When necessary, sediment was carefully removed under the microscope with a soft brush or a wet tooth pick. This resulted in the retention of 159 pieces bearing compelling traces of manufacture and use, unmodified or marginally modified shell fragments probably used as beads, and modified and unmodified lumps of iron-rich rock and sediments, possibly used to extract ocher powder. The retained artifacts were examined at magnifications between ×4 and ×40, and photographed with a motorized Leica Z6 APOA microscope equipped with a Leica Application Suite (LAS) and Multifocus module, and Leica Map DCM 3D computer software. The Multifocus module enables the acquisition of extended depth of field images. Once the digital images had been complete for different heights, algorithms in the software compile them into a single composite images that significant extends the depth of field, and provides clarity in viewing the entire object. The selected areas of one Conus shell were scanned using a Sensofar Sneox scanning confocal microscope with a ×20 objective. The resulting files were analyzed with Mountains 7.2 software. For further details on the analytical protocols for beads, osseuous artifacts, and ocher see Supplementary Note 4 and the references therein. A full description of all osseous artifacts, beads, and used ocher will be reported elsewhere, but Fig. 3 shows examples of each of these artifact types from PYS excavation, and Supplementary Figure 19 gives an overview of their distribution through the sequence. Phytolith analysis Seventeen sediment samples from the continuous stratigraphic column described in SM3 were processed for phytolith analysis. Of these, the lower six samples were barren. We followed extraction protocols employed on Middle Stone Age sites from adjacent countries [66] and modern topsoils [67] . The procedure included sieving, drying, deflocculating, acid/base treatment, and sequential density separation by manipulating the specific gravity of sodium polytungstate. Aliquot mounting was with “Entellan New,” which allowed for microscopic inspection (×40) and 3D rotation before drying. The average count per slide was 238 phytoliths. The inferential baseline was grounded on East African phytoliths from plants and soils [68] , [69] . Preservation was adequate for morphometric analysis and type identification. Mollusk analysis Macro marine molluskan remains were identified and counted by Patrick Faulkner using comparative modern reference collections. Since no evidence for subsistence on these was found prior to Layer 6, they will be reported in detail elsewhere. PYS is an open-roofed cave with substantial input from the external environment. The paleoenvironmental samples recovered from PYS contained terrestrial mollusk fauna representing the area in and immediately outside the cave over a long time period [70] . There is no evidence that any of these species have been transported to the site through natural or anthropogenic processes. Excluding large marine shells that form part of the archeological record, the aquatic component of the assemblage is extremely small and is less significant than that seen in faunas from the modern coastal forests on Zanzibar. As a result, transport by fluvial activity or regular flooding of the area can be ruled out. The diverse community of snails could not have been sustained in a closed cave environment but would have required continual external input in the form of leaf litter and the snails themselves or their shells. The non-marine mollusk record from PYS therefore offers a long record of the local environment through time. Tetrapod analysis The zooarchaeological analysis of PYS osseous remains took place in 2012 (Trench 3) and 2014 (Trench 4) and produced a database of 5256 identified specimens (Number of Identified Specimens, NISP). A total of 6.4 kg of bone was excavated from Trench 3 and 14.7 kg from Trench 4. The Trench 4 study included both taxonomic identification and taphonomic analysis, but microfauna were not analyzed in Phase 1 due to time constraints. In Trench 3, microfauna were identified to a very general level (e.g., “Muridae”). Initial sorting of faunal remains created up to three categories: first, maximally identifiable (maxID) specimens include teeth and those bones that preserve at least one articular surface and/or key landmark, enabling identification to element and usually to taxon or at least taxonomic group (e.g., “bird,” “small carnivore”). MaxID specimens were identified in all contexts in both trenches. Second, minimally identifiable (minID) bones include limb shafts and axial fragments that can generally be identified at least to carcass size; these were identified in nine high-priority contexts from Trench 4, in order to obtain a sample for taphonomic analysis. Third, nonidentified (NID) bones were separated from minID specimens and weighed in these selected contexts. On average across all contexts in Trench 4, 10% of the assemblage was maximally identifiable. When minID specimens identified in nine selected contexts were included the average identification rate rose to 37%. Taxonomic identifications were made on the basis of extensive reference collections housed at the National Museums of Kenya (Nairobi) Osteology Unit. Calculations of the minimum number of individuals (MNI) were made using the resulting database following completion of this analysis and took into account specimen laterality, size, and where relevant, age estimates. It should be stressed that limb shafts were only studied in selected contexts and therefore could not be used to calculate the minimum number of elements (MNE) or the resulting MNI values for layers or phases, as is standard practice in contexts where density-mediated attrition has occurred. It is therefore possible that MNI estimates will be too low in some instances. Stable carbon and oxygen isotope analysis of mammalian tooth enamel Stable isotope analysis of mammalian tissues has frequently been used to assess the diets and ecologies of East African fossil fauna [71] , [72] , [73] . This work primarily relies on the distinction between the C 3 - or C 4 -photosynthetic pathways at the base of East African foodwebs. In the context of tropical and sub-tropical forest ecologies, this distinction can be used to assess the degree of faunal reliance on C 3 forest resources as opposed to C 4 plant resources available in open habitats, with C 4 plants being enriched in 13 C relative to C 3 plants [74] , [75] , [76] . This distinction is further enhanced by the “canopy effect” whereby vegetation growing under a closed forest canopy is strongly depleted in 13 C (with correspondingly lower measured δ 13 C) due to low light and the presence of large amounts of respired CO 2 [77] , [78] . This results in the tissues of animals consuming forest vegetation, as well as forest herbivores, having lower δ 13 C values than animals pending some, or all, of their time consuming open-habitat foodstuffs e.g. [79] . Stable oxygen isotope measurements from mammalian enamel can yield further paleoecological information about water and food [80] , [81] . Given a constant source of water, plant water δ 18 O will primarily reflect the impacts of relative humidity on leaf water evapotranspiration, with decreasing humidity resulting in increased δ 18 O values [82] , [83] , [84] . In a tropical or sub-tropical setting, increased forest cover, and the resulting shade and increased humidity, will lead to decreased evapotranspiration and therefore decreased δ 18 O, especially on the forest floor [79] . As faunal tooth enamel δ 18 O primarily reflects water and food-water δ 18 O, herbivores feeding and drinking in forests can be expected to have lower enamel δ 18 O than those feeding in open, irradiated areas. This is complicated by physiological and behavioral variables [85] . Nevertheless, animals consuming plants and water in a shaded, forested setting will broadly reflect the corresponding lower levels of evapotranspiration in their enamel δ 18 O. Stable carbon and oxygen isotope analysis of faunal tooth enamel excavated from the various archeological Phases at PYS was undertaken in order to directly assess the diets and ecologies of animals being exploited by humans living at the site at different points in time. This should, in turn, provide information regarding fluctuations in the degree of forest cover surrounding PYS in the past. Faunal enamel samples were taken from all available PYS Layers. A broad selection of species was sampled for each Layer based on availability. Where possible, up to five members of each species/genus were sampled per layer grouping (Supplementary Data 1 ). Faunal samples were identified to species and/or genus level using the substantial reference collection available at the National Museums of Kenya, Nairobi. The full list of faunal samples and tooth identifications analyzed in this study are shown in Supplementary Data 1 . Air-abrasion was used to remove any adhering detrital material from the teeth or tooth fragments to be studied. Gentle abrasion with a diamond-tipped drill was performed along the full length of the buccal surface of the tooth or tooth fragment in order to maximize the period of formation represented by the resulting isotopic analysis. The resulting enamel powder was pretreated using standard, published protocols in order to remove any organic or secondary carbonate contaminates. This consisted of a wash in 1.5% sodium hypochlorite for 60 min, followed by three rinses in purified H 2 O. A volume of 0.1 M acetic acid was then added for 10 min prior to another three rinses in purified H 2 O [86] , [87] . 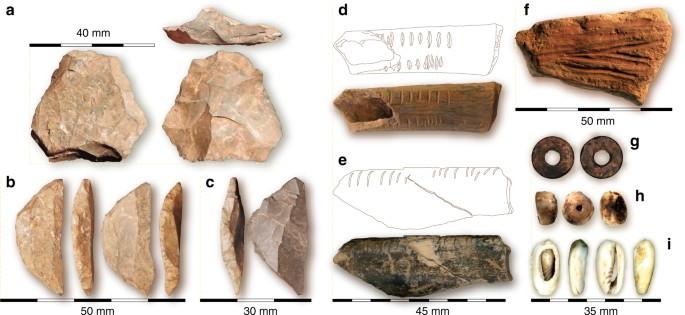Fig. 2 Selected artifacts from PYS.aLevallois core from Layer 11.bTwo backed lithic artifacts from Layer 11.cBacked lithic artifact from Layer 3.dNotched bone from Layer 8.eNotched bone from Layer 9.fOcher crayon from Layer 10.gOstrich eggshell bead from Layer 8.hConusshell bead from Layer 16.iGastropod shell bead from Layer 4 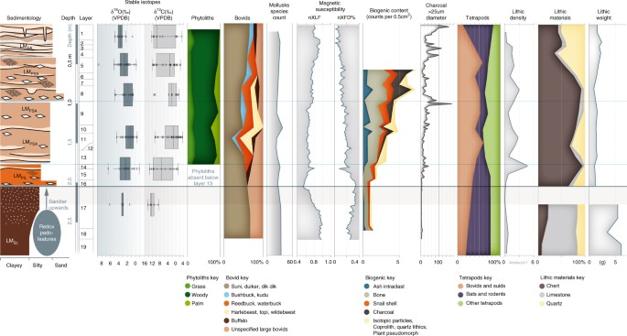Fig. 3 The palaeoenvironmental and human occupation proxies from PYS. From left to right: Sedimentology (LM(SC) sandy clayey loam, LM(PS) pebbly sandy loam, LM(PSA) pebbly sandy ashy loam, LM(SA) sandy ashy loam); Depth; Layer divisions; Box and whisker plots of stable oxygen and carbon isotope values of mammalian teeth; Phytoliths, showing the proportion of grass, palm, and woody taxa; Percentage of different bovids in Minimum Number of Individuals (MNI); Terrestrial mollusk rarefied species count; Magnetic susceptibility (XLF and XFD%); Biogenic content of micromorphology thin sections; Microcharcoal abundance; Proportions of selected faunal groups as a percentage of total tetrapod MNI; Lithic density; Lithic material types; Lithic weight (mean debitage weight) Gases were evolved from the treated samples using 100% Phosphoric Acid. t δ 13 C and δ 18 O of the resulting gases was measured using a Thermo Gas Bench 2 connected to a Thermo Delta V Advantage Mass Spectrometer at the Division of Archeological, Geographic and Environmental Sciences Bradford University. δ 13 C and δ 18 O measurements from samples were compared against international standards (NBS 19 and CO-9) registered by the International Atomic Energy Agency (five of each for a run of 60). Replicate analysis of in-house OES and MERCK standards (six of each for a run of 60) suggests that machine measurement error is c . ±0.1‰ for δ 13 C and ±0.2‰ for δ 18 O. Analysis of variance (ANOVA) tests were performed on faunal enamel δ 13 C and δ 18 O to determine whether these isotopic parameters differed between groups of stratigraphic layers. The stratigraphic layers were grouped based on meaningful chronological and stratigraphic divisions as follows: 1–3, 4–6, 7–9, 10–12, 13–16, and 17. Where variance was found to be significant following ANOVA testing, a post-hoc Tukey pair-wise comparison was performed in order to determine which layer groupings were significantly different from each other in terms of δ 13 C and δ 18 O. All statistical analyses were conducted using the free program R software [88] . Data availability The authors declare that all data supporting the findings of this study are available upon request from the authors. The artifacts and faunal remains from the Panga ya Saidi excavation are curated in the National Museum of Kenya, Nairobi, under the site code PYS and the suffixes 10, 11, and 13 (denoting the year of excavation).